Identification of genes involved in the biology of atypical teratoid/rhabdoid tumours usingDrosophila melanogaster Atypical teratoid/rhabdoid tumours (AT/RT) are malignant brain tumours. Unlike most other human brain tumours, AT/RT are characterized by inactivation of one single gene, SMARCB1 . SMARCB1 is a member of the evolutionarily conserved SWI/SNF chromatin remodelling complex, which has an important role in the control of cell differentiation and proliferation. Little is known, however, about the pathways involved in the oncogenic effects of SMARCB1 inactivation, which might also represent targets for treatment. Here we report a comprehensive genetic screen in the fruit fly that revealed several genes not yet associated with loss of snr1 , the Drosophila homologue of SMARCB1. We confirm the functional role of identified genes (including merlin , kibra and expanded , known to regulate hippo signalling pathway activity) in human rhabdoid tumour cell lines and AT/RT tumour samples. These results demonstrate that fly models can be employed for the identification of clinically relevant pathways in human cancer. Atypical teratoid/rhabdoid tumours (AT/RT) are highly malignant human brain tumours mainly affecting young children. Even though intensive multimodal therapy has resulted in some improvement [1] , prognosis for most children with AT/RT remains dismal. The vast majority of AT/RT shows biallelic inactivating mutations of the SMARCB1 gene (also known as hSNF5/INI1) [2] , while other recurrent genetic alterations are lacking [3] , [4] , [5] . SMARCB1 is a member of the SWI/SNF chromatin remodelling complex, which is evolutionarily highly conserved and plays a critical role in the epigenetic control of cell differentiation and proliferation [6] . Little is known, however, on molecular mechanisms through which SMARCB1-deficiency drives oncogenesis [7] . Only few targetable genes and pathways like Cyclin D1 (ref. 8 ) and Hedgehog-Gli [9] have been linked to SMARCB1 deficiency and broad functional screens for genes and pathways associated with SMARCB1 loss have not been feasible. Drosophila melanogaster allows for genetic and functional studies at a rate unmatched by current mammalian models [10] , [11] , [12] . We therefore established a Drosophila melanogaster modifier screen in order to identify pathways involved in the phenotype associated with ubiquitous or glial-specific knockdown of snr1 , the fly homologue of SMARCB1 . Here we show that hippo signalling is involved in the phenotype associated with snr1 knockdown and also plays a role in the biology of human AT/RT. Silencing of snr1 results in phenotypic changes in the fly Silencing of snr1 messenger RNA (mRNA) expression using the Gal4-UAS system ( Supplementary Fig. 1 ) resulted in decreased Snr1 protein levels upon ubiquitous or glial-specific snr1 knockdown, respectively ( Fig. 1a,e ). While ubiquitous silencing of snr1 mRNA expression inevitably resulted in larval death (L2 stage), glial-specific silencing of snr1 was associated with death at the pupal stage of development. The Gal4-UAS system thus represents a suitable model for high throughput screening of genes resulting in a positive or negative shift of the lethal phenotypes, that is, genes worsening or weakening the effect of snr1 silencing. Phenotypically, ubiquitous ( Fig. 1b–d ) and glial-specific snr1 knockdown ( Fig. 1f–h ) resulted in increased volume of the larval fly brain, which was associated with increased proliferation ( Fig. 1d,h ). Proliferating cells stained positive for the neural precursor marker Prospero or the neuroblast marker Deadpan, but not for the neuronal marker Elav or the glial marker Repo ( Supplementary Fig. 2 ), suggesting that snr1 is essential for the regulation of neural precursor proliferation and the development of the fly brain. A snr1 null mutant [ snr1 01319 ; Supplementary Fig. 3 ) was associated with a more severe phenotype (embryonal death), impeding the use of this strain in a modifier screen. 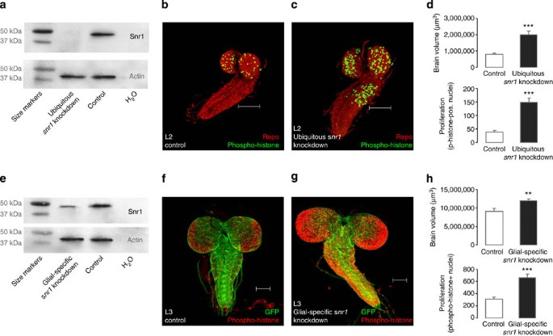Figure 1: Phenotype uponsnr1knockdown inDrosophila melanogaster. Phenotype upon ubiquitous (a–d) and glial-specific (e–h)snr1knockdown. (a) Western blot confirming absence of Snr1 protein upon ubiquitoussnr1knockdown (whole L2 larvae). As compared withtubGal4 control (b) knockdown ofsnr1is associated with increased proliferation and brain volume of the L2 larval brain (c). Representative confocal images of L2 brains showing glial nuclei (Repo; red) and proliferating cells (phospho-histone; green, scale bars, 100 μm). (d) Ubiquitoussnr1knockdown increases volume (1,998,912±223,600 μm3versus 790,910±64,220 μm3, mean±s.e.m.,N=15, ***P<0.001, two-tailedt-test) as well as proliferation (149±15 versus 38±6 phospho-histone-positive nuclei; mean±s.e.m.,N=15,P<0.001, two-tailedt-test) of the larval L2 brain. (e) Western blot confirming reduction of Snr1 protein upon glial-specificsnr1knockdown (whole brains, L3 larvae). As compared with control (repoGal4>UAS-mCD8-GFP, (f) knockdown ofsnr1is associated with increased proliferation and brain volume of the L3 larval brain (g). Representative confocal images of L3 brains showing glial cells (UAS-mCD8-GFP expression driven by repo-Gal4 (green) as well as proliferating cells (phospho-histone; red, scale bars, 100 μm). Upon glial-specificsnr1knockdown, brain volume (11,950,934±575,200 μm3versus 9,090,203±793,600 μm3, mean±s.e.m.,N=15, **P<0.01, two-tailedt-test) as well as proliferation (656±58 versus 310±33 phospho-histone-positive nuclei; mean±s.e.m., N=15, ***P<0.001, two-tailedt-test) is also increased. Figure 1: Phenotype upon snr1 knockdown in Drosophila melanogaster . Phenotype upon ubiquitous ( a – d ) and glial-specific ( e – h ) snr1 knockdown. ( a ) Western blot confirming absence of Snr1 protein upon ubiquitous snr1 knockdown (whole L2 larvae). As compared with tub Gal4 control ( b ) knockdown of snr1 is associated with increased proliferation and brain volume of the L2 larval brain ( c ). Representative confocal images of L2 brains showing glial nuclei (Repo; red) and proliferating cells (phospho-histone; green, scale bars, 100 μm). ( d ) Ubiquitous snr1 knockdown increases volume (1,998,912±223,600 μm 3 versus 790,910±64,220 μm 3 , mean±s.e.m., N =15, *** P <0.001, two-tailed t -test) as well as proliferation (149±15 versus 38±6 phospho-histone-positive nuclei; mean±s.e.m., N =15, P <0.001, two-tailed t -test) of the larval L2 brain. ( e ) Western blot confirming reduction of Snr1 protein upon glial-specific snr1 knockdown (whole brains, L3 larvae). As compared with control ( repo Gal4>UAS-mCD8-GFP, ( f ) knockdown of snr1 is associated with increased proliferation and brain volume of the L3 larval brain ( g ). Representative confocal images of L3 brains showing glial cells (UAS-mCD8-GFP expression driven by repo-Gal4 (green) as well as proliferating cells (phospho-histone; red, scale bars, 100 μm). Upon glial-specific snr1 knockdown, brain volume (11,950,934±575,200 μm 3 versus 9,090,203±793,600 μm 3 , mean±s.e.m., N =15, ** P <0.01, two-tailed t -test) as well as proliferation (656±58 versus 310±33 phospho-histone-positive nuclei; mean±s.e.m., N=15, *** P <0.001, two-tailed t -test) is also increased. Full size image Shift of lethal phenotype on modifier screen Crossing snr1 knockdown flies with strains expressing specific RNA interference shifted the L2 lethal phenotype associated with ubiquitous snr1 knockdown to later stages of development in 9 out of 1,015 screened candidate genes ( Fig. 2a , Supplementary Data 1 , see Supplementary Data 2 for complete list of screened small interfering RNAs (siRNAs)), suggesting that these genes are required for the lethal phenotype associated with snr1 loss in Drosophila melanogaster . Of note, silencing of merlin resulted in the most pronounced shift in phenotype (64% hatched animals). The lethal phenotype associated with glial-specific snr1 knockdown was shifted to later stages of development in 60 out of 1,015 screened candidate genes, whereas silencing of five genes led to aggravation of the phenotype and death at the larval or embryonal stage ( Fig. 2a , Supplementary Data 1 ). Gene ontology (GO) categories significantly overrepresented among the identified candidate genes included GO:0005488 (binding; χ 2 test P <0.0000001), GO:0043167 (ion binding; P <0.05) and GO:0001071 (nucleic acid binding transcription factor activity; P <0.05) ( Supplementary Fig. 4 ). Genes associated with a shift to later stages of development not only involved Cyclin D and cubitus interruptus , whose human homologues CCND1 and GLI1 are well recognized to drive the growth of SMARCB1 -deficient malignant rhabdoid tumours [13] , [14] , but also kibra and expanded , whose products (together with Merlin) form a complex representing a key upstream regulator of the hippo pathway [15] , [16] , [17] . Because no other pathway was represented with more genes, the role of hippo signalling was examined in more detail. Glial-specific knockdown of kibra and expanded did not alter the efficiency of snr1 knockdown ( Fig. 2b ), but resulted in reduction of the increased brain volume observed upon snr1 knockdown ( Fig. 2c ). Furthermore, as compared with wild-type controls, mRNA expression of merlin , kibra and expanded was significantly upregulated upon both ubiquitous ( Fig. 2d ) and glial-specific snr1 knockdown ( Fig. 2e ). While yorkie was not among the genes associated with a shift to later stages of development, Yorkie activity (as assessed by mRNA expression of target genes CyclinE and DIAP1 ) was increased upon snr1 knockdown. Additional ubiquitous knockdown of merlin resulted in a significant decrease of the elevated DIAP1 and CyclinE expression levels ( Fig. 2f,g ). Glial-specific double knockdown of snr1 and expanded in repo Gal4> snr1 > ex dsRNA flies resulted in increased expression of DIAP1 , while repo Gal4> snr1 > kibra dsRNA flies showed decreased expression of CyclinE and unaltered DIAP1 expression ( Supplementary Fig. 5 ). 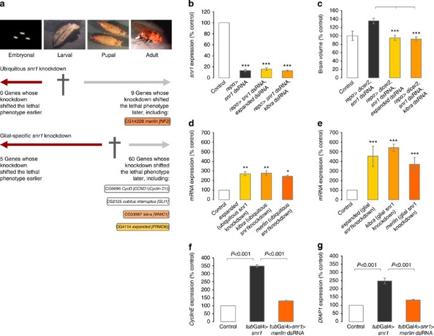Figure 2: Modifier screen inDrosophila melanogaster. (a) Crossingsnr1knockdown flies with strains expressing specific RNA interference (RNAi) shifted the L2 lethal phenotype associated with ubiquitoussnr1knockdown to later stages of development in 9 out of 1,015 screened candidate genes includingmerlin. Crossing ofsnr1knockdown flies with strains expressing specific RNAi shifted the pupal lethal phenotype associated with glial-specificsnr1knockdown to later stages of development in 60 out of 1,015 screened candidate genes including hippo signalling regulatorskibraandexpanded. (b) Quantitative RT–PCR confirming efficient silencing ofsnr1expression uponsnr1knockdown alone (14%±2%) and upon additional knockdown ofexpanded(16%±2%) orkibra(13%±1%), respectively (mean±s.e.m.,N=3, ***P<0.001 versus Control, analysis of variance (ANOVA) followed byt-test with Bonferroni correction) (c). As compared with glial-specificsnr1knockdown alone, which resulted in increased volume of the L3 larval brain as compared with control (136%±6%), additional knockdown ofexpandedorkibracaused reversal of the brain phenotype with significant reduction in brain volume (95%±6% and 93%±5%, respectively, mean±s.e.m.,N=8–15, ***P<0.001, ANOVA followed byt-test with Bonferroni correction). (d) mRNA expression ofmerlin,kibraandexpandedwas significantly upregulated upon ubiquitoussnr1knockdown as well as (e) glial-specificsnr1knockdown (mean±s.e.m.,N=4 each, ***P<0.001 versus control, **P<0.01 versus control, *P<0.05 versus control, ANOVA followed byt-test with Bonferroni correction). Ubiquitoussnr1knockdown resulted in increased expression of Yorkie activity markersCyclinE(f) andDIAP1(g). Additional ubiquitous knockdown of merlin resulted in a significant decrease of the elevatedDIAP1andCyclinEexpression levels (mean±s.e.m.,N=3,P-values determined by ANOVA followed byt-test with Bonferroni correction). Figure 2: Modifier screen in Drosophila melanogaster . ( a ) Crossing snr1 knockdown flies with strains expressing specific RNA interference (RNAi) shifted the L2 lethal phenotype associated with ubiquitous snr1 knockdown to later stages of development in 9 out of 1,015 screened candidate genes including merlin . Crossing of snr1 knockdown flies with strains expressing specific RNAi shifted the pupal lethal phenotype associated with glial-specific snr1 knockdown to later stages of development in 60 out of 1,015 screened candidate genes including hippo signalling regulators kibra and expanded . ( b ) Quantitative RT–PCR confirming efficient silencing of snr1 expression upon snr1 knockdown alone (14%±2%) and upon additional knockdown of expanded (16%±2%) or kibra (13%±1%), respectively (mean±s.e.m., N =3, *** P <0.001 versus Control, analysis of variance (ANOVA) followed by t -test with Bonferroni correction) ( c ). As compared with glial-specific snr1 knockdown alone, which resulted in increased volume of the L3 larval brain as compared with control (136%±6%), additional knockdown of expanded or kibra caused reversal of the brain phenotype with significant reduction in brain volume (95%±6% and 93%±5%, respectively, mean±s.e.m., N =8–15, *** P <0.001, ANOVA followed by t -test with Bonferroni correction). ( d ) mRNA expression of merlin , kibra and expanded was significantly upregulated upon ubiquitous snr1 knockdown as well as ( e ) glial-specific snr1 knockdown (mean±s.e.m., N =4 each, *** P <0.001 versus control, ** P <0.01 versus control, * P <0.05 versus control, ANOVA followed by t -test with Bonferroni correction). Ubiquitous snr1 knockdown resulted in increased expression of Yorkie activity markers CyclinE ( f ) and DIAP1 ( g ). Additional ubiquitous knockdown of merlin resulted in a significant decrease of the elevated DIAP1 and CyclinE expression levels (mean±s.e.m., N =3, P -values determined by ANOVA followed by t -test with Bonferroni correction). Full size image Taken together, these results suggest that genes whose products regulate the hippo signalling pathway are essential for the phenotype associated with snr1 loss in Drosophila melanogaster . Hippo signalling has a role in human rhabdoid tumour cells The hippo pathway plays a key role in the development and regulation of organ size [18] . It is composed of a core kinase cascade that is regulated by multiple upstream inputs (for review see refs. 15 , 17 ). Hippo activation leads to phosphorylation of Yorkie, which in turn results in cytoplasmatic retention and suppression of its transcriptional activity. Inactivating mutations of pathway elements as well as overexpression of Yorkie have been shown to delay or block the differentiation of neuroepithelial cells [19] . Increasing evidence suggests that disruption of hippo signalling might also play a role in human cancer [20] , [21] . In SMARCB1 -deficient rhabdoid tumour cell lines BT16, A204 and G401, we found NF2 , WWC1 and FRMD6 , the homologues of merlin , kibra and expanded , to be expressed ( Fig. 3a–c ). Transient silencing of NF2 , WWC1 and FRMD6 expression in BT16 cells was effective on mRNA ( Fig. 3d–f ) and protein level ( Supplementary Fig. 6 ). Transient silencing resulted in reduced proliferative activity on methylthiazolyldiphenyl-tetrazolium bromide (MTT) and BrdU assay, while cytotoxicity was unaltered ( Fig. 3g–i , Supplementary Fig. 7 ). Comparable results were obtained in rhabdoid tumour cell lines A204 and G401 ( Supplementary Fig. 8 ). Importantly, triple knockdown of NF2 , WWC1 and FRMD6 in BT16 cells did not result in a significant additive effect on proliferative activity (MTT assay) as compared with single knockdown of NF2 , WWC1 and FRMD6 ( Fig. 3k ). In mammals, the Yorkie homologue Yes-associated protein 1 (YAP1) represents the main effector of the hippo pathway and exerts its effects by forming nuclear complexes with co-activators of the TEAD family [22] , [23] . Expression of YAP1 protein and phosphorylated YAP1 protein could be demonstrated in all three rhabdoid tumour cell lines examined ( Supplementary Fig. 9a,b ). The drug verteporfin suppresses the oncogenic activity of YAP by disruption of TEAD-YAP complexes [24] , [25] . At concentrations that have been shown to specifically inhibit TEAD-YAP interactions in sensitive cells (that is, 1–5 μM) [24] , verteporfin attenuated proliferation ( Fig. 3j ) as well as migration ( Supplementary Fig. 9f ) of SMARCB1 -deficient rhabdoid tumour cells. Because these data suggest that the YAP/TEAD complex might play a role in these settings, YAP1 knockdown experiments were performed. In rhabdoid tumour cell line G401, knockdown of YAP1 resulted in a significant reduction of proliferation. This effect was less pronounced in A204 and BT16 cells ( Supplementary Fig. 9 ) Of note, YAP1 protein expression was markedly lower in G401 cells ( Supplementary Fig. 9 ), suggesting that long half-life of the YAP1 protein could be at least partly responsible for the absence of significant effects in BT16 and A204. 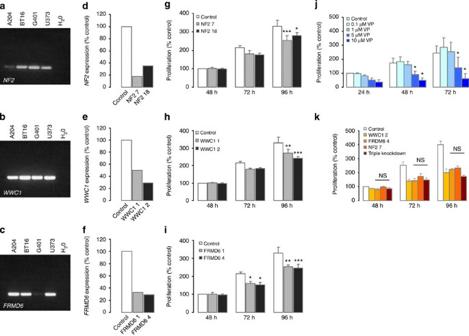Figure 3: Functional role of hippo signalling in human rhabdoid tumour cells. RT–PCR confirming mRNA expression of (a)NF2, (b)WWC1and (c)FRMD6in rhabdoid tumour cell lines BT16, A204 and G401 as well as in U373 cells (control). In BT16 cells, silencing ofNF2,WWC1andFRMD6using two different siRNAs effectively reduced mRNA expression (d–f) and resulted in significantly reduced proliferative activity (MTT assay) as compared with controls (non-target siRNA,g–i, means±s.e.m.,N=3, ***P<0.001 versus control, **P<0.01, *P<0.05 versus control, analysis of variance (ANOVA) followed byt-test with Bonferroni correction). (j) Dose-dependent effect of verteporfin (VP) on proliferative activity in BT16 cells showing significantly reduced proliferation after 48 h and 72 h of incubation as compared with control (means±s.e.m., N=3, *P<0.05 versus control, ANOVA followed byt-test with Bonferroni correction). (k) Triple knockdown ofWWC1,FRMD6andNF2in BT16 cells did not result in a significant additive effect on proliferative activity (MTT assay) as compared with single knockdown ofNF2,WWC1andFRMD6(means±s.e.m.,N=3, ANOVA followed byt-test with Bonferroni correction). Figure 3: Functional role of hippo signalling in human rhabdoid tumour cells. RT–PCR confirming mRNA expression of ( a ) NF2 , ( b ) WWC1 and ( c ) FRMD6 in rhabdoid tumour cell lines BT16, A204 and G401 as well as in U373 cells (control). In BT16 cells, silencing of NF2 , WWC1 and FRMD6 using two different siRNAs effectively reduced mRNA expression ( d – f ) and resulted in significantly reduced proliferative activity (MTT assay) as compared with controls (non-target siRNA, g – i , means±s.e.m., N =3, *** P <0.001 versus control, ** P <0.01, * P <0.05 versus control, analysis of variance (ANOVA) followed by t -test with Bonferroni correction). ( j ) Dose-dependent effect of verteporfin (VP) on proliferative activity in BT16 cells showing significantly reduced proliferation after 48 h and 72 h of incubation as compared with control (means±s.e.m., N=3, * P <0.05 versus control, ANOVA followed by t -test with Bonferroni correction). ( k ) Triple knockdown of WWC1 , FRMD6 and NF2 in BT16 cells did not result in a significant additive effect on proliferative activity (MTT assay) as compared with single knockdown of NF2 , WWC1 and FRMD6 (means±s.e.m., N =3, ANOVA followed by t -test with Bonferroni correction). Full size image Taken together, these results suggest that hippo signalling is involved in the biology of SMARCB1 -deficient rhabdoid tumour cells and could represent a potential therapeutic target. YAP1 is overexpressed and plays a prognostic role in AT/RT On gene expression profiling of AT/RT, mRNA expression of NF2 , WWC1 , FRMD6 as well as YAP1 was present, WWC1 and YAP1 being highly overexpressed as compared with medulloblastomas as well as non-neoplastic control tissues ( Fig. 4a , Supplementary Fig. 10 , Supplementary Data 3 ). In an independent series of 34 AT/RT samples obtained from the European Rhabdoid Tumour Registry (EU-RHAB), for which detailed clinical information was available ( Supplementary Data 4 ), YAP1 protein expression was present in the majority of tumours ( Fig. 4b ) and associated with shorter progression-free survival and overall survival ( Fig. 4c,d ). Taken together, these results suggest that hippo signalling is also perturbed in SMARCB1-deficient AT/RT. 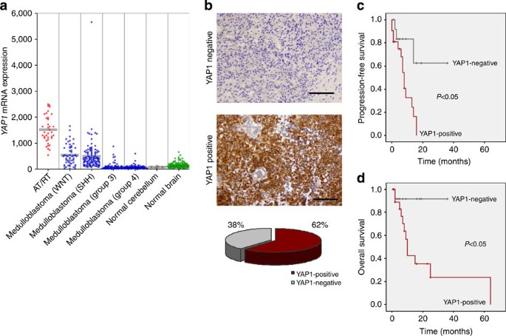Figure 4: Expression and prognostic role of hippo pathway transcriptional co-activator YAP1 in AT/RT. (a) Gene expression profiling (Affymetrix U133plus2.0 arrays) of 37 AT/RT showing increasedYAP1mRNA expression as compared with 442 medulloblastomas of all four molecular subgroups (WNT, SHH, Group 3, Group 4) as well as samples from normal cerebellum (N=9) and normal CNS tissues (N=169). Analysis of variance was used to test whether there is a significant differential expression between the groups shown in the plots (P=1.6 × 10−115). (b) Using immunohistochemistry on formalin‐fixed paraffin‐embedded tissue samples, YAP1 protein expression (brown, below) was present in 21 out of 34 AT/RT examined (62%). Scale bars, 100 μm. On Kaplan–Meyer analysis, progression‐free survival (c) and overall survival (d) were both shorter in children showing YAP1 protein expression (P<0.05, log‐rank test). Figure 4: Expression and prognostic role of hippo pathway transcriptional co-activator YAP1 in AT/RT. ( a ) Gene expression profiling (Affymetrix U133plus2.0 arrays) of 37 AT/RT showing increased YAP1 mRNA expression as compared with 442 medulloblastomas of all four molecular subgroups (WNT, SHH, Group 3, Group 4) as well as samples from normal cerebellum ( N =9) and normal CNS tissues ( N =169). Analysis of variance was used to test whether there is a significant differential expression between the groups shown in the plots ( P =1.6 × 10 −115 ). ( b ) Using immunohistochemistry on formalin‐fixed paraffin‐embedded tissue samples, YAP1 protein expression (brown, below) was present in 21 out of 34 AT/RT examined (62%). Scale bars, 100 μm. On Kaplan–Meyer analysis, progression‐free survival ( c ) and overall survival ( d ) were both shorter in children showing YAP1 protein expression ( P <0.05, log‐rank test). Full size image Drosophila melanogaster models play an increasing role in tumour research [12] and have been employed to recapitulate certain aspects of glioblastoma [11] , [26] . In contrast to glioblastomas and the majority of paediatric brain tumours, which represent multiple subgroups with diverse genetic and epigenetic background [27] , [28] , [29] , recurrent genetic alterations in AT/RT are mainly restricted to the SMARCB1 gene, which is evolutionarily highly conserved [3] , [4] , [5] . Thus, AT/RT represent a tumour entity ideally suited for modelling in Drosophila . Indeed, siRNA-mediated knockdown of snr1 , the fly homologue of SMARCB1 resulted in a lethal phenotype, allowing for high throughput screens of genes functionally involved in snr1 deficiency. We also note that knockdown of snr1 results in increased volume of the larval brain and proliferation of neural precursors, suggesting that snr1 is not only involved in wing patterning, abdomen development and sustained adult viability [30] , [31] , but also plays an important role in the development of the fly nervous system. Interestingly, this phenotype was observed upon both ubiquitous and glial-specific snr1 knockdown. The latter finding might well be explained by re-programming of snr1 deficient repo expressing glial cells towards a more immature phenotype, but could also suggest that functional snr1 in glial cells is required for the regulation of brain volume and neural proliferation. In our fly model, the functional role of a large number of genes not yet associated with snr1 loss could be demonstrated, including members of the notch and hippo signalling pathways, which regulate cell–cell communication and neural development [19] . The finding that ubiquitous knockdown of merlin reverted the lethal phenotype associated with snr1 knockdown is unexpected, because it suggests a detrimental role for NF2 in the context of SMARCB1 deficiency. A detrimental role of Merlin under conditions of snr1 deficiency is further supported by the finding that mRNA expression levels of both DIAP1 and CyclinE , genes known to inhibit apoptosis and to support proliferation, were downregulated upon merlin silencing. Of note, DIAP1 and CyclinE are well established markers for Yorkie activity in fly tissues [18] . Merlin forms a complex with Kibra and Expanded, which has been shown to be an important upstream regulator of hippo signalling [16] , [32] . The fact that silencing of kibra and expanded also shifted the lethal phenotype observed upon glial-specific snr1 knockdown and caused reversal of the CNS phenotype, supports an unfavourable role of this complex under conditions of reduced snr1 expression. This view is further substantiated by the fact that knockdown of the respective human homologues NF2 , WWC1 and FRMD6 resulted in decreased proliferation of SMARCB1 -deficient rhabdoid tumour cells. The finding that triple knockdown of these genes did not result in an additive effect on proliferation further supports a functional role of the hippo pathway (rather than individual genes) in SMARCB1 deficiency. Activation of Yorkie, the main effector of hippo signalling, drives proliferation of glial cells [33] . Upon both ubiquitous and glial-specific knockdown of snr1 , we found expression of DIAP1 and CyclinE to be upregulated, suggesting that Yorkie activity under these conditions is increased [18] . In humans, overexpression of the Yorkie homologue YAP1 has been demonstrated in malignant brain tumours and linked to more aggressive behaviour in glioblastoma [34] . The observation that YAP1 was overexpressed in AT/RT as compared with other malignant pediatric brain tumours and associated with shorter survival suggests a role of hippo signalling in the biology of AT/RT. It remains to be elucidated how WWC1, FRMD6 and NF2 dysfunction is related to YAP1 overexpression under conditions of SMARCB1 deficiency. One possibility involves interactions with other signalling pathways. Indeed, in Drosophila melanogaster , crosstalk of hippo signalling with other pathways including Wnt, Tgfβ and Notch has been shown to regulate stem cell fate [35] . In vertebrates, Kibra (mainly expressed in brain and kidney, the main sites of malignant rhabdoid tumours) is essential for the full activation of aurora kinases [36] , which have been shown to be essential for survival of SMARCB1 -deficient rhabdoid tumour cells [37] . In Drosophila melanogaster , functional Snr1 has been shown to be critical for the actions of chromatin remodelling complex member Brahma [38] . Of note, Brahma recently also has been shown to interact with hippo signalling [39] , [40] , suggesting a connection between Brahma, Snr1 and hippo signalling via possibly more than one signalling route. In conclusion, a large number of novel genes functionally involved in the detrimental effects of snr1 deficiency could be identified in Drosophila melanogaster . Among those, genes of the hippo signalling pathway play a role in the biology and possibly therapy of AT/RT. Fly work All crosses were performed at 25 °C and raised on cornmeal-yeast agar. Strains used were as follows: w 1118 , repo -Gal4, repo 4.3-Gal4, Tb, tub Gal80 (all kindly provided by Christian Klämbt), tub Gal4>lysGFP and snr1 01319 mutant (both provided by Bloomington Drosophila Stock Center, Bloomington, IN), UAS- dicer2 (kindly provided by Jürgen Knoblich). UAS- snr1 dsRNA, UAS- expanded dsRNA, UAS- kibra dsRNA, UAS- merlin dsRNA were all obtained from VDRC Stock Center (Vienna, Austria). All dsRNA lines used for the modifier screen were obtained from VDRC and the Harvard Drosophila stock collection ( Supplementary Table 2 ). Candidate genes for the modifier screen were chosen based on the availability of dsRNA lines and known expression in the nervous system of Drosophila melanogaster (based on searches of Flybase; www.flybase.org ). The fly strain with the genotype UAS-snr1 dsRNA , repo -Gal4>UAS-mCD8GFP; repo -Gal4/Tb, tub Gal80 and the strain with the genotype UAS-snr1 dsRNA ; tub -Gal4lysGFP/Tb, tub Gal80 were used for the modifier screen. Here, Gal4 mediated expression is blocked by Gal80 protein. If these flies are crossed against wild-type flies, Gal80 is lost. The glial strain dies as pupae (25 °C), the ubiquitous strain dies at the L2 larval stage (22 °C). When UAS -snr1 dsRNA ,repo -Gal4>UAS-mCD8GFP ; repo -Gal4/Tb, tub Gal80 flies are crossed to flies carrying UAS-dsRNA constructs, snr1 and genes are silenced in glial cells in the F1 generation. The progeny of such crosses were kept at 25 °C and scored for a shift in the lethal phenotype. To score the shift in lethality the percentage of hatched flies was calculated by counting the number of adults and comparing with the whole number of pupae ( N =47 (38–63); median; quartiles). To be classified as modifier gene, at least 10% of flies needed to be shifted in three independent experiments ( Supplementary Data 1 ). When UAS- snr1 dsRNA; tub -Gal4lysGFP/Tb, tub Gal80 flies are crossed to flies carrying UAS-dsRNA constructs, snr1 and genes are silenced in all cells in the next generation. The progeny of such crosses were kept at 22 °C and scored for a shift in the lethal phenotype. The strain UAS- dicer2 ;UAS- snr1 dsRNA, repo -Gal4>UAS-mCD8GFP; repo -Gal4/Tb, tub Gal80 was used for the quantification of L3 brain volume upon glial-specific double knockdown of snr1 and expanded or snr1 and kibra , respectively. Quantification of larval fly brain volume For quantification of larval brain volume in Drosophila melanogaster , images were taken using Laser Scanning microscope (710 Zeiss, Zeiss, Oberkochen, Germany). For digital analysis, the LSM Image Browser from Zeiss was utilized. Area of the larval brain of each single plane was scaled and multiplied with single plane thickness. Summation of all measured single planes resulted in total brain volume. Immunohistochemistry of the larval fly brain Fixation of L3 larvae brains was carried out with 3.7% formalin. Specimens were mounted in Vectashield (Vector Laboratories, Burlingame, CA). Mouse anti-Repo (1:5), mouse anti-Elav (1:4) and mouse anti-Prospero antibodies (1:4) were obtained from the Developmental Studies Hybridoma Bank (Iowa City, IA). Rabbit anti-phospho-histone H3 (Ser10; 1:500) was obtained from Millipore (Darmstadt, Germany). Guinea-pig anti-Deadpan (1:500) was kindly provided by Jürgen Knoblich. Cy5 (1:200, Dianova, Hamburg, Germany), Cy2 (1:100, Sigma-Aldrich, München, Germany) and Cy3 (1:200, Sigma-Aldrich) were used as secondary antibodies. Fluorescently labelled specimens were analysed using a Zeiss LSM 710 microscope. Quantification of proliferation in the larval fly brain For image analysis, the open source software CellProfiler [41] was used. Briefly, z-stack images were converted into a single plane image by generating a maximum intensity projection of the z-planes. The maximum intensity projection was then submitted to Cell Profiler 2.0.0 (revised r11710) to enumerate phospho-histone stained cells. The module ColorToGray (splitting the different colour channels into grey pictures) was applied where multi-colour pictures were submitted. Furthermore, the modules ImageMath (enhancing background to noise ratio) and IndentifyPrimaryObjects (× 20 pictures: identify and count stained objects between 5 and 50 pixel; × 40 pictures: identify and count stained objects between 10 and 50 pixel in diameter) were used. For × 20 pictures Otsu Global algorithm and for × 40 pictures RidlerCalvard Adaptive algorithm was used to distinguish between background and signal. Intensity and shape were applied in order to separate and draw dividing lines between clumped objects. After each IdentifyPrimaryObjects module a PauseCellProfiler module was added to visually control the result. Quantitative RT–PCR For fly samples, total RNA was isolated from L3 larval brain (glial-specific knockdown) or whole larvae (ubiquitous knockdown) with GenElute (Sigma-Aldrich). cDNA was generated using the High capacity cDNA Reverse Transcription Kit (Applied Biosystems, Darmstadt, Germany) following the manufacturer’s instructions. Quantitative RT–PCR was performed in triplicate using SYBR Green (Life Technologies, Darmstadt, Germany) or TaqMan Gene Expression Assays for monoplex reaction following the manufacturer’s instructions. The transcription levels of mRNA were analysed using comparative Ct method. The following primers were obtained for SYBR green from MWG-Eurofins (Ebersberg, Germany): kibra (5′-GAAAGGAGCTGGCACAAGTC; 3′-TGGTCCTTATGGAGGTCAGC) and Act5c (5′ GAGCGCGGTTACTCTTTCAC; 3′-ACTTCTCCAACGAGGAGCTG). The following primers were obtained for TaqMan Gene Expression Assays (Life Technologies): snr1 (Dm02147905_g1; FAM-labelled), expanded (Dm01841942_g1; FAM-labelled), merlin (Dm01813975_g1; FAM-labelled) and Act5c (Dm02361909_s1; FAM-labelled). For expression analysis of Yorkie activity markers DIAP1 and CyclinE , the following primers were obtained for TaqMan Gene Expression Assays (Life Technologies): DIAP1 (Dm02362595_s1; FAM‐labelled) and CyclinE (Dm01807603_g1; FAM‐labelled). Protein expression of Snr1 For western blot analysis, protein from total larvae extracts (ubiquitous snr1 knockdown) or larval brains (glial-specific snr1 knockdown) were mixed with 4 × SDS sample buffer, boiled and separated by electrophoresis on 12% polyacrylamide SDS gels. Pre-stained protein ladder was used as a size standard for molecular mass determination (Abcam, Cambridge, UK). Gels were electroblotted onto polyvinylidene difluoride membranes using a wet blotting apparatus (Bio-Rad, München, Germany). The blot was incubated with rabbit anti-SNF5 antibody in 0.5% powdered milk (1:500, Abcam) for 90 min. Subsequently, the blot was incubated for 1 h with Anti-Rabbit IgG (whole molecule)–Peroxidase (1:30,000, Sigma-Aldrich). All steps were proceeded at room temperature. Visualization of Snr1 was performed by chemiluminescence (Luminata Forte Western HRP substrate, Millipore). Uncropped images of the western blots used in Fig. 1 are provided as Supplementary Fig. 11 . Cell lines Human rhabdoid tumour cells BT16 (brain), A204 (liver) and G401 (kidney) were obtained from ATCC (Manassas, VA). Profiling of the cell lines for genetic alterations of the SMARCB1 region on 22q was done by FISH and sequencing as described previously [4] . While no larger deletions were detectable in BT16 cells, heterozygous and homozygous deletions of the SMARCB1 region were present in A204 and G401 cells, respectively. On sequencing, heterozygous SMARCB1 deletions were detectable in BT16 (177_178delGA) and A204 (543-544delTC) causing premature stop codons. SMARCB1 immunohistochemistry of formalin-fixed paraffin-embedded rhabdoid tumour cell pellets (anti-SMARCB1, 1:200; #612110, BD Biosciences, Heidelberg, Germany) confirmed lack of nuclear SMARCB1 immunoreactivity in all three cell lines. Cell culture conditions Cells were cultured in Dulbecco’s modified Eagle’s minimal essential medium (DMEM; PAA, Linz, Austria). For A204 and G401 cell media was supplemented with 10% fetal calf serum (FCS-Gold, PAA) and 10% penicillin/streptomycin (PAA). BT16 cell media was supplemented with 16.6% fetal calf serum (Life Technologies), 10% L -glutamine (Life Technologies) and 10% penicillin/streptomycin (P/S; PAA). Cells were incubated under standard conditions (37 °C in a 5% CO 2 humidified atmosphere) as described previously [42] . RT–PCR For human samples, after RNA isolation (Maxwell® 16 LEV simplyRNA Tissue Kit on Maxwell 16 Instrument, Promega, Mannheim, Germany) RNA was transcribed into cDNA (High Capacity cDNA Reverse Transcription Kit, Life Technologies) according to standard protocols. Expression of genes of interest was tested by PCR amplification (HotStarTaq Plus DNA Polymerase, Qiagen, Hilden, Germany). Primer were obtained from MWG-Eurofins (WWC1: 5′-CGCTGACGGAGAGGTTAAAG-3′; 5′-GCTGAAGTGGAGGAGTCCAG-3′/FRMD6: 5′-CTGGTCCAGGTTTGTGACCT-3′; 5′-ATTGGTCGATACCCTTGCTG-3′/NF2: 5′-GGGATGAAGCTGAAATGGAA-3′/5′-AGGAGATCTTGGGGGTCAGT-3′). Quantitative RT–PCR For human samples, after RNA isolation and reverse transcription (see above), mRNA expression levels were examined using the following TaqMan Gene Expression Assays (Life Technologies) (SMARCB1 (Hs00268260_m1; FAM-labelled), WWC1 (Hs00392086_m1; FAM-labelled), FRMD6 (Hs00378563_m1; FAM-labelled) and NF2 (Hs00966302_m1; FAM-labelled)) and normalized to glyceraldehyde-3-phosphate dehydrogenase (GAPDH) expression using primers GAPDH-fwd 5′-ACCCACTCCTCCACCTTTGAC-3′, GAPDH-rev 5′-CATACCAGGAAATGAGCTTGACAA-3′, and GAPDH-probe 5′-CTGGCATTGCCCTCAACGACCA-3′ (MWG Eurofins). All experiments were performed in triplicate. Protein expression in human rhabdoid tumour cells Western blots were carried out using 90 μg of total protein from cell lysates. For sample preparation, a 4 × SDS sample buffer was added, followed by boiling at 95 °C for 5 min. Protein separation was conducted with electrophoresis in 12% polyacrylamide/SDS gels. For electroblotting cellulose membranes (Whatman, Dassel, Germany) in combination with a wet blotting apparatus (Bio-Rad) were used. The membrane was incubated with NF2 antibody (1:200; sc-331, Santa Cruz, Dallas, TX), WWC1 antibody (1:500; kindly provided by Dirk Oliver Wennmann and Joachim Kremerskothen (Department of Molecular Nephrology, University Hospital Münster, Germany)), FRMD6 antibody (1:2,000; ab171745, Abcam), YAP1 antibody (1:1,000; #4912, Cell Signaling, Danvers, MA) or YAP1-Phospho antibody (1:10,000; ab76252, Abcam), respectively, as well as a β-actin antibody (1:10,000; A5441, Sigma-Aldrich) as house-keeping gene in 0.5% powdered milk for 90 min. As secondary antibodies, anti-rabbit IgG peroxidase (1:10,000, Sigma-Aldrich) or anti-mouse IgG peroxidase (1:10,000, Sigma-Aldrich) in 0.5% powdered milk were used. During the whole detection process with YAP1-phospho antibody bovine serum albumin was used instead of powdered milk. The incubation time was 90 min. Visualization of the proteins was performed by chemoluminescence (Luminata Forte Western HRP substrate, Millipore). Gene silencing siRNA oligonucleotides were obtained from Qiagen [Hs_WWC1_1 FlexiTube siRNA (SI03185035), Hs_WWC1_2 FlexiTube siRNA (SI04234489), Hs_FRMD6_1 FlexiTube siRNA (SI03169572), Hs_FRMD6_4 FlexiTube siRNA (SI04351466), Hs_NF2_7 FlexiTube siRNA (SI02664137), Hs_NF2_18 FlexiTube siRNA (SI04949959), Hs_YAP1_6 FlexiTube siRNA (SI04438637) and Hs_YAP1_8 FlexiTube siRNA (SI04438651)]. As transfection control served a non-silencing negative control (Ctrl_AllStars_1 (SI03650318); Qiagen). 5 × 10 5 (A204, BT16 and G401) cells in 500 μl antibiotic-free media were plated on 24-well dishes and transfected with siRNA at a concentration of 10 nM using 4.5 μl HiPerFect Transfection Reagent (Qiagen). For triple knockdown experiments, siRNA oligonucleotides Hs_WWC1_2 FlexiTube siRNA (SI04234489), Hs_FRMD6_4 FlexiTube siRNA (SI04351466), Hs_NF2_7 FlexiTube siRNA (SI02664137) and the non-silencing negative control (Ctrl_AllStars_1 (SI03650318) from Qiagen were used. 5 × 10 5 cells of BT16 cell line in 500 μl antibiotic-free media were plated on 24-well dishes and transfected with (1) siRNA for single knockdown of WWC1 , NF2 or FRMD6 (10 nM) and the non-silencing negative control siRNA (20 nM), (2) a combination of all three siRNAs for triple knockdown of WWC1 , FRMD6 and NF2 (10 nM each), (3) non-silencing siRNA (30 nM) as a negative control. To each sample 13.5 μl HiPerFect Transfection Reagent (Qiagen) was added. MTT assay Cellular viability and growth were assessed by MTT assay. Cells were either incubated in the presence of varying concentrations of verteporfin (Visudyne, Novartis, Basel, Switzerland), or siRNA knockdown of the hippo pathway components NF2 , WWC1 and FRMD6 . The MTT assay was performed as described previously [42] . Experiments were independently performed in triplicates and for each condition, a number of eight wells were used. For verteporfin experiments, cell suspensions (10,000 cells per 100 μl) were seeded into 96-well plates. Twenty-four hours later, medium was exchanged against 100 μl of medium containing different concentrations of verteporfin (0.001–10 μM) was added. Proliferation was assessed using a MTT assay as described earlier [43] . For evaluation of WWC1 , NF2 and FRMD6 knockdown and triple knockdown effects, knockdown was conducted as described above and cells were subsequently seeded into 96-well plates at 10,000 cells per 60 μl. Cell viability was measured after 48, 72 or 96 h. BrdU assay Proliferation was assessed by (colorimetric) BrdU assay (Roche, Mannheim, Germany) according to manufacturer’s protocol. After siRNA knockdown of the hippo pathway components WWC1 , NF2 and FRMD6 , 10,000 cells per well were seeded out into a 96-well plate and incubated for 48, 72 and 96 h. Incubation time with BrdU labelling solution was 4 h and for anti-BrdU-POD working solution 90 min. Experiments were independently performed in triplicates and for each condition, a number of three wells were used. Cytotoxicity assay Cytotoxicity was assessed by CytoTox-Glo Cytotoxicity Assay (Promega). Cells were transfected with siRNA as described above and 10,000 cells were seeded out per 96-well followed by an incubation time of 96 h. Cytotoxicity was measured according to manufacturer’s protocol. Experiments were independently performed in triplicates and for each condition a number of three wells were used. Migration assay Cell migration kinetics were conducted in CIM-Plate 16 (Roche) and recorded by the X-Celligence instrument (Roche) for less than 24 h period, depending on the cell line. For BT16, a number of 75,000 cells per well were seeded out in serum-free media, but with different verteporfin concentrations (1, 5 and 10 μM) into the top chamber. Preincubation of CIM-Plate 16 containing 160 μl serum-supplemented media in the lower chamber was carried out for 1 h in the CO 2 incubator at 37 °C. Migration was monitored every 15 min over several hours. Gene expression profiling All mRNA expression data of human samples have been generated by Affymetrix U133plus2.0 arrays. Gene expression data come from public sources deposited in GEO ( http://www.ncbi.nlm.nih.gov/geo ; GSE10327 (ref. 44 ), GSE37418 (ref. 45 ), GSE12992 (ref. 46 ), GSE3526 (ref. 47 ), GSE35493 (ref. 48 )) or have been generated at the German Cancer Research Center DKFZ in Heidelberg. The MAS5.0 algorithm of the GCOS program (Affymetrix, Santa Clara, CA) was used for normalization of the expression data. All data have been analysed using the R2 program for analysis and visualization of microarray data ( http://R2.amc.nl ). AT/RT samples for YAP1 protein expression Formalin-fixed paraffin-embedded archival samples of 34 AT/RT were retrieved from the archives of the Institute of Neuropathology, Münster. Patients had been enrolled in the EU-RHAB from which detailed clinical information was obtained. EU-RHAB has received ethical committee approval (Ethics committee of the University Hospital Münster, 2009-532-f-S) and parents had given informed consent for scientific use of the archival samples. All cases were primary tumours. The diagnosis was confirmed neuropathologically according to current WHO criteria. The diagnostic workup also included immunohistochemical staining for SMARCB1 protein [49] as well as staining for SMARCA4/BRG1 (ref. 50 ). YAP1 immunohistochemistry For YAP1 immunohistochemistry, a mouse antiserum against YAP1 (dilution 1:50; sc-10119, Santa Cruz Biotechnology) was used. The specificity of this antiserum for YAP1 has been confirmed previously [51] . Immunohistochemistry was performed on de-paraffinized and rehydrated sections without pretreatment using the 3,3′-diaminobenzidine method on an automated staining system (Auto Stainer Link 48, DAKO, Glostrup, Denmark) according to the manufacturer’s protocol. Sections were counterstained with haematoxylin. Staining was rated as 0 (absent) or 1 (present). Statistics Quantification of brain volume and proliferating cells were statistically evaluated by two-tailed t -test. Proliferative effects of gene knockdown were statistically evaluated using analysis of variance followed by t -test with Bonferroni correction for post hoc comparison. GraphPad PRISM software was used (Graph Pad Software, San Diego, CA) for these analyses. Kaplan–Meyer analysis of survival and progression-free survival data was done using IBM SPSS Statistics software (release 21.0). Comparison between groups was done by Log-Rank test. How to cite this article : Jeibmann, A. et al . Identification of genes involved in the biology of atypical teratoid/rhabdoid tumours using Drosophila melanogaster . Nat. Commun. 5:4005 doi: 10.1038/ncomms5005 (2014).